Interconnect-free parallel logic circuits in a single mechanical resonator In conventional computers, wiring between transistors is required to enable the execution of Boolean logic functions. This has resulted in processors in which billions of transistors are physically interconnected, which limits integration densities, gives rise to huge power consumption and restricts processing speeds. A method to eliminate wiring amongst transistors by condensing Boolean logic into a single active element is thus highly desirable. Here, we demonstrate a novel logic architecture using only a single electromechanical parametric resonator into which multiple channels of binary information are encoded as mechanical oscillations at different frequencies. The parametric resonator can mix these channels, resulting in new mechanical oscillation states that enable the construction of AND, OR and XOR logic gates as well as multibit logic circuits. Moreover, the mechanical logic gates and circuits can be executed simultaneously, giving rise to the prospect of a parallel logic processor in just a single mechanical resonator. The concept of encoding multiple signals with different frequencies was originally pioneered in optical fibre networks to increase their capacity [1] , [2] , [3] . To achieve this, wavelength division multiplexing (WDM) was developed, which enables a single optical fibre to operate as if it were a bundle of fibres. State-of-the-art WDM can enable more than a 1,000 different wavelengths of light to propagate in parallel through a single fibre, yielding a dramatic increase in signal throughput in an optical fibre network. Conceptually, WDM can be regarded as not addressing real space, that is, the choice of a particular optical fibre, but rather as addressing frequency space, that is, the choice of wavelength in a given optical fibre. On the basis of this principle, here, we demonstrate the Boolean logic analogue [4] where binary information is not encoded in physically distinct devices, but is instead encoded as different oscillation frequencies in a single device—the increasingly common electromechanical resonator [5] , [6] . This novel approach allows a single device to not only operate as if it were a fully integrated logic circuit but also to operate as a parallel logic processor enabling the simultaneous execution of multiple Boolean functions where crucially all interconnects have been eliminated. Device The GaAs/AlGaAs-based mechanical resonator used in this study is shown and described in Figures 1a and 1b , and has a fundamental mode at f 0 = ω 0 /2 π =155,702 Hz with a quality factor Q =140,000 ( Fig. 1c and Methods) [7] . The piezoelectric effect in the GaAs/AlGaAs heterostructure can enable electrical actuation and detection of mechanical motion as well as the parametric amplification via force constant modulation [8] , [9] , [10] . 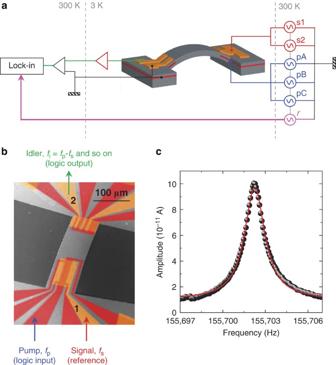Figure 1: The electromechanical parametric resonator. (a) A schematic of the experimental setup where the mechanical resonator is in the geometry of a doubly clamped beam (grey) with a length, width and thickness of 260, 84, and 1.35 μm, respectively, and it hosts an out-of-plane oscillation mode. The mechanical oscillator has Schottky Au-electrodes (orange) located above both clamping points, below which a 2DEG is located (red). Application of a.c. bias to either the 2DEG or the Au-electrodes can trigger both harmonic and parametric resonances where the mechanical motion is monitored by detecting in either a lock-in amplifier or a spectrum analyser the motion-induced piezovoltage, which is amplified by an on-chip amplifier (red triangle) and a room temperature transimpedance amplifier (black triangle). In all cases, the signals s1 and s2 are applied to the large Au-electrode with a 50 μVrmsactuation amplitude and the pumps pA, pB and pC are applied to the 2DEG with 40 mVrmsactuation amplitude where the referenceris used for the lock-in measurements. (b) A false-colour scanning electron microscopic image of the electromechanical resonator where the pump (logic input), signal excitation (to functionalize logic operations) and the idler (logic output) are marked. (c) The electromechanical resonance (dots) measured via the lock-in amplifier and fitted with a harmonic oscillator response (line). Figure 1: The electromechanical parametric resonator. ( a ) A schematic of the experimental setup where the mechanical resonator is in the geometry of a doubly clamped beam (grey) with a length, width and thickness of 260, 84, and 1.35 μm, respectively, and it hosts an out-of-plane oscillation mode. The mechanical oscillator has Schottky Au-electrodes (orange) located above both clamping points, below which a 2DEG is located (red). Application of a.c. bias to either the 2DEG or the Au-electrodes can trigger both harmonic and parametric resonances where the mechanical motion is monitored by detecting in either a lock-in amplifier or a spectrum analyser the motion-induced piezovoltage, which is amplified by an on-chip amplifier (red triangle) and a room temperature transimpedance amplifier (black triangle). In all cases, the signals s1 and s2 are applied to the large Au-electrode with a 50 μV rms actuation amplitude and the pumps pA, pB and pC are applied to the 2DEG with 40 mV rms actuation amplitude where the reference r is used for the lock-in measurements. ( b ) A false-colour scanning electron microscopic image of the electromechanical resonator where the pump (logic input), signal excitation (to functionalize logic operations) and the idler (logic output) are marked. ( c ) The electromechanical resonance (dots) measured via the lock-in amplifier and fitted with a harmonic oscillator response (line). Full size image Among the 12 independent electrical contacts, a single two-dimensional electron gas (2DEG) contact is used for binary information input with a frequency around 2 f 0 , and the gate located directly above (gate 1) is used for injecting an excitation around f 0 . Henceforth, these excitations are termed pump and signal, respectively, in analogy with frequency conversion in optical parametric amplifiers [11] . The signal can directly excite a mechanical oscillation and is necessary for functionalizing logic operations. In contrast, the pump cannot directly excite mechanical motion as its amplitude is below the parametric resonance threshold [7] . However, the interaction between signal and pump results in the excitation of mechanical motion as shown below. Within the resonance bandwidth, multiple oscillations at different frequencies can be simultaneously excited by injecting multiple pumps with slightly different frequencies. In all cases, the motion was electrically detected via gate 2, that is, this gate is used for the readout of Boolean functions as shown in Figure 1b . Mechanical idler generation Parametric frequency conversion has an essential role in the execution of logic functions in this architecture and its operation is first described here [12] , [13] . A pump with fixed frequency, f p =2 f 0 , is injected into the 2DEG, while a signal at frequency f s = f 0 + δ , where δ is a variable, is applied to gate 1. 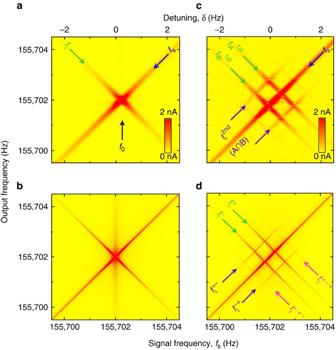Figure 2: The mechanical idler dynamics. (a) The response of the mechanical oscillator measured via the lock-in amplifier withfp=2f0+Δ where Δ=0 Hz andfs=f0+δreveals the fundamental modefsand the idlerfi=f0−δ. (b) The corresponding theoretical response generated from equation (9) (Methods). (c) The response of the mechanical oscillator measured via the lock-in amplifier, withfpA=2f0+Δ andfpB=2f0−Δ where Δ=0.5 Hz, andfs=f0+δreveals, in addition tofs, the two first-order idlersandand two second-order idlersthat can be used to implement mechanical logic gates. (d) The corresponding numerical simulation except equation (9) is modified to include two pumps, and all the higher order idlers are labelled (Methods). In all cases, the experimental response is broader than the numerical simulations because of an experimental resolution band width (RBW) of 50 mHz. The frequency response measured via gate 2 is shown in Figure 2a as a function of f s and the corresponding theoretical response is shown in Figure 2b (Methods). In addition to the input signal (blue arrow), an additional oscillation with a negative slope (green arrow) is observed. This excitation arises because of mixing between f p and f s resulting in the creation of an idler at f i = f p − f s = f 0 − δ , thus demonstrating mechanical parametric frequency conversion for the first time ( Supplementary Note 1 and Supplementary Figure S1 ). Figure 2: The mechanical idler dynamics. (a ) The response of the mechanical oscillator measured via the lock-in amplifier with f p =2 f 0 +Δ where Δ=0 Hz and f s = f 0 + δ reveals the fundamental mode f s and the idler f i = f 0 − δ . ( b ) The corresponding theoretical response generated from equation (9) (Methods). ( c ) The response of the mechanical oscillator measured via the lock-in amplifier, with f pA =2 f 0 +Δ and f pB =2 f 0 −Δ where Δ=0.5 Hz, and f s = f 0 + δ reveals, in addition to f s , the two first-order idlers and and two second-order idlers that can be used to implement mechanical logic gates. ( d ) The corresponding numerical simulation except equation (9) is modified to include two pumps, and all the higher order idlers are labelled (Methods). In all cases, the experimental response is broader than the numerical simulations because of an experimental resolution band width (RBW) of 50 mHz. Full size image Logic gates To demonstrate the AND (∩) operation, two pump excitations with frequency f pA =2 f 0 +Δ and f pB =2 f 0 −Δ with fixed detuning Δ are injected into the 2DEG, which correspond to binary inputs A and B, respectively, where the absence (presence) of the pump yields the binary input 0 (1). The frequency response measured via gate 2 and shown in Figure 2c (along with the corresponding theoretical response in Fig. 2d ) now reveals not only the above first-order idlers f iA = f 0 +Δ− δ and f iB = f 0 −Δ− δ (green arrows) corresponding to the two pumps but also two second-order idlers (purple arrows). The second-order idlers arise because of mixing between the first-order idlers f iA and f iB , and the two pumps f pA and f pB , resulting in f pA − f iB = f 0 +2Δ+ δ and f pB − f iA = f 0 −2Δ+ δ (Methods). It should be emphasized that the second-order idlers can only be created when the two pumps pA and pB are active, thus enabling the execution of the A∩B logic gate where the absence (presence) of the idlers corresponds to the binary output 0 (1). Next, to demonstrate the OR ( ∪ ) operation, the mechanical resonator is injected with two signals at f s1 = f 0 +Δ+ δ and f s2 = f 0 −Δ+ δ , which results in the reference vibrations being excited by both s1 and s2 ( Supplementary Note 2 and Supplementary Figure S2 ). 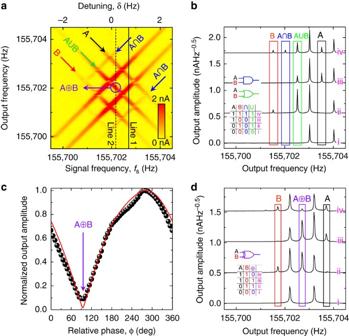Figure 3: Mechanical logic gates. (a) The mechanical resonator's response measured via the lock-in amplifier with two signal excitations atfs1=f0+Δ+δandfs2=f0−Δ+δand two pump excitations atfpA=2f0+Δ andfpB=2f0−Δ where Δ=0.5 Hz. Using this response, an ∩ gate can be realized by any second-order idler (blue arrows), the∪gate can be realized via the degenerate first-order idler (green arrow) and the⊕gate can be realized via the degenerate idler at exactlyfr=f0(purple circle). (b) Two-bit binary input channels A and B can be encoded viafpAandfpBwhere the ∩ and∪logic gates can be realized by measuring the response of the mechanical resonator along the line 1 inaas a function of pump A and B, while both signal excitations are active. The resulting response measured via a spectrum analyser with a RBW of 25 mHz reveals both ∩ and∪gates in parallel in a single mechanical resonator. (c) The⊕gate can also be realized via the degenerate idler at exactlyfr=f0(purple circle ina) by varying the phase difference between s1 and s2, which can lead to both constructive and destructive interference. The destructive interference can be used to realize a⊕logic gate whenφ=94° where the dots are from the experimental measurement and the line is the result of a numerical simulation (Methods). (d) The⊕gate is demonstrated along line 2 inaatfr=f0by measuring the response of the mechanical resonator in a spectrum analyser with RBW=25 mHz as a function of pA and pB when the phase difference between s1 and s2 is 94° with an on/off ratio of 10:1. All the spectra are offset for clarity and are numbered (roman numerals) to correlate with the numbered truth combinations in their corresponding truth tables where the various inputs and gates have been colour coded. The complete set of idlers created when all the signals and pumps are activated is shown in Figure 3a . Activating only f pA yields two first-order idlers f 0 − δ (green arrow) and f 0 − δ +2Δ (black arrow A). Activating only f pB yields f 0 − δ −2Δ (red arrow B) and f 0 − δ (green arrow). From these measurements, it is seen that the f 0 − δ idler can be excited by either pump A or pump B, which enables the realization of the A ∪ B gate. The mechanical frequency response obtained at a fixed signal frequency (along line 1 in Fig. 3a ) as a function of pump excitation is shown in Figure 3b and it clearly demonstrates the AND and OR operation. It should be emphasized that the two logic outputs can be obtained in parallel with only a single device in contrast to conventional logic devices where only sequential operation is available. Figure 3: Mechanical logic gates. ( a ) The mechanical resonator's response measured via the lock-in amplifier with two signal excitations at f s1 = f 0 +Δ+ δ and f s2 = f 0 −Δ+ δ and two pump excitations at f pA =2 f 0 +Δ and f pB =2 f 0 −Δ where Δ=0.5 Hz. Using this response, an ∩ gate can be realized by any second-order idler (blue arrows), the ∪ gate can be realized via the degenerate first-order idler (green arrow) and the ⊕ gate can be realized via the degenerate idler at exactly f r = f 0 (purple circle). ( b ) Two-bit binary input channels A and B can be encoded via f pA and f pB where the ∩ and ∪ logic gates can be realized by measuring the response of the mechanical resonator along the line 1 in a as a function of pump A and B, while both signal excitations are active. The resulting response measured via a spectrum analyser with a RBW of 25 mHz reveals both ∩ and ∪ gates in parallel in a single mechanical resonator. ( c ) The ⊕ gate can also be realized via the degenerate idler at exactly f r = f 0 (purple circle in a ) by varying the phase difference between s1 and s2, which can lead to both constructive and destructive interference. The destructive interference can be used to realize a ⊕ logic gate when φ =94° where the dots are from the experimental measurement and the line is the result of a numerical simulation (Methods). ( d ) The ⊕ gate is demonstrated along line 2 in a at f r = f 0 by measuring the response of the mechanical resonator in a spectrum analyser with RBW=25 mHz as a function of pA and pB when the phase difference between s1 and s2 is 94° with an on/off ratio of 10:1. All the spectra are offset for clarity and are numbered (roman numerals) to correlate with the numbered truth combinations in their corresponding truth tables where the various inputs and gates have been colour coded. Full size image To implement the XOR ( ⊕ ) gate, we exploit the interference between the two idlers along f 0 − δ by simply adjusting the relative phase φ between s1 and s2. At an appropriate value of φ , the f 0 − δ idler can be completely cancelled at f s = f 0 when both pumps A and B are active as shown in Figure 3c , which enables the realization of the A ⊕ B gate as a function of pump excitation (along line 2 in Fig. 3a ) as shown in Figure 3d . The realization of a universal electromechanical logic gate in a single device with AND, OR and XOR functions can enable the construction of any other logic gate. Logic circuits Beyond the implementation of fundamental two-bit logic gates, we also investigate the prospect of multibit logic circuits in a single mechanical resonator. 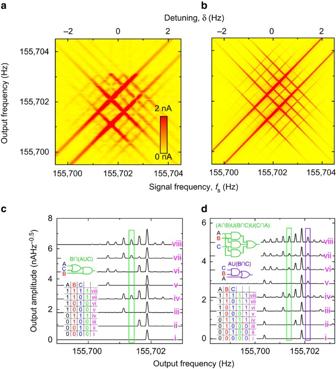Figure 4: Multibit mechanical logic circuits. (a) The response of the mechanical resonator measured via the lock-in amplifier with two signal excitations atfs1=f0+Δ+δandfs2=f0−Δ+δand three pumpsfpA=2f0+Δ,fpB=2f0−Δ andfpC=2f0+2Δ where Δ=0.5 Hz. (b) The corresponding numerical simulation except equation (9) is modified to include three pumps and two signals (Methods). (c) The 3-bit B∩(A∪C) logic circuit is constructed with the two second-order idlersfpB−(fpA−fs) andfpB−(fpC−fs) where Δs1=Δs2=0.5 Hz, ΔpA=0.25 Hz, ΔpB=−0.25 Hz and ΔpC=0.75 Hz. (d) The A∪(B∩C) and (A∩B)∪(B∩C)∪(C∩A) logic circuits are constructed in parallel from first and second-order idlersfpA=fs,fpB−(fpC−fs) and three second-order idlersfpA−(fpB−fs),fpB−(fpC−fs) andfpC−(fpA−fs), respectively, with Δs1=0.5 Hz, Δs2=−1 Hz, ΔpA=0.25 Hz, ΔpB=−0.25 Hz and ΔpC=0.75 Hz. In both cases, the mechanical parametric resonator was sampled via a spectrum analyser with an RBW=12.5 mHz. All the spectra are offset for clarity and are numbered (roman numerals) to correlate with the numbered truth combinations in their corresponding truth tables where the various inputs and circuits have been colour coded. To do this, a third pump is injected into the system at f pC =2 f 0 +2Δ, which is used to encode a third-bit labelled as C. The resulting response of the system measured as above via gate 2 as a function of f s is shown in Figure 4a along with the corresponding theoretical response in Figure 4b (Methods). Figure 4: Multibit mechanical logic circuits. ( a ) The response of the mechanical resonator measured via the lock-in amplifier with two signal excitations at f s1 = f 0 +Δ+ δ and f s2 = f 0 −Δ+ δ and three pumps f pA =2 f 0 +Δ, f pB =2 f 0 −Δ and f pC =2 f 0 +2Δ where Δ=0.5 Hz. ( b ) The corresponding numerical simulation except equation (9) is modified to include three pumps and two signals (Methods). ( c ) The 3-bit B∩(A ∪ C) logic circuit is constructed with the two second-order idlers f pB −( f pA − f s ) and f pB −( f pC − f s ) where Δ s1 =Δ s2 =0.5 Hz, Δ pA =0.25 Hz, Δ pB =−0.25 Hz and Δ pC =0.75 Hz. ( d ) The A ∪ (B∩C) and (A∩B) ∪ (B∩C) ∪ (C∩A) logic circuits are constructed in parallel from first and second-order idlers f pA = f s , f pB −( f pC − f s ) and three second-order idlers f pA −( f pB − f s ), f pB −( f pC − f s ) and f pC −( f pA − f s ), respectively, with Δ s1 =0.5 Hz, Δ s2 =−1 Hz, Δ pA =0.25 Hz, Δ pB =−0.25 Hz and Δ pC =0.75 Hz. In both cases, the mechanical parametric resonator was sampled via a spectrum analyser with an RBW=12.5 mHz. All the spectra are offset for clarity and are numbered (roman numerals) to correlate with the numbered truth combinations in their corresponding truth tables where the various inputs and circuits have been colour coded. Full size image To demonstrate a multibit logic circuit, we implement the sequence B∩(A ∪ C), where A, B and C are the binary input channels at f pA , f pB and f pC , respectively. This logic circuit can be decomposed as B∩A and B ∪ C, which can be mathematically represented by two second-order idlers f pB −( f pA − f s ) and f pB −( f pC − f s ), where f s is either due to s1 or s2. To achieve maximum fidelity for this logic circuit, the idlers must only intersect with each other and their visibility will be maximized at f 0 . Rewriting the signal and pump excitations as f s1 = f 0 +Δ s1 , f s2 = f 0 +Δ s2 , f pA =2 f 0 +Δ pA , f pB =2 f 0 +Δ pB and f pC =2 f 0 +Δ pC can enable these boundary conditions to be expressed as 0=Δ pB −Δ pA +Δ s(1 or 2) and 0=Δ pB −Δ pC +Δ s(1 or 2) , where Δ pA ≠Δ pB ≠Δ pC . From these expressions, the detunings for the signal and pump excitations that lead to 100% fidelity for the B∩(A ∪ C) logic circuit can be extracted, and the resulting circuit is executed in Figure 4c . Using a similar analytical approach, various 3-bit logic circuits can be constructed in parallel including (A∩B) ∪ (B∩C) ∪ (C∩A), that is, the majority gate which is shown in Figure 4d ( Supplementary Figure S3 for additional circuits). All logic operations including multibit logic circuits can be reproduced by numerical simulations, thus enabling more advanced logic circuits to be easily designed (Methods). A generalized formulism to implement multibit logic circuits for arbitrary Boolean functions will be reported elsewhere. The first programmable computer was pioneered in a mechanical architecture almost two centuries ago [14] . However, mechanical computation was rendered obsolete with the advent of the transistor [15] , which gave rise to an electrical binary-unit (bit) for Boolean logic [4] . With the recent emergence of electromechanical resonators [5] , [6] , the concept of a mechanical computer has been revived as this offers the tantalizing prospect of low power consumption [16] . In spite of some recent experimental effort, a universal electromechanical logic gate based on Boolean algebra has remained beyond reach [7] , [17] , [18] , [19] , [20] . The parametric frequency conversion demonstrated here not only permits the realization of all the primary logic gates in an electromechanical resonator for the first time [16] , [18] , [19] , [20] , [21] but it also enables multibit logic circuits to be executed in a single mechanical resonator as well as providing an architecture in which parallel logic circuits can be easily constructed. Consequently, a mechanical computer based on these concepts offers the prospect of unrivalled integration density, low power consumption [7] , [16] and potentially high speed, as information does not have to be passed between multiple transistors as in conventional sequential logic circuits. Moreover, this concept contributes significantly to the beyond transistor-based computation debate [22] . To translate this proof-of-principle prototype into a more practical device, both room temperature and atmospheric operation is a necessary prerequisite. Although the present device can operate at room temperature [23] , the viscous damping present at atmospheric pressure degrades its performance. The effects of viscous damping could be reduced by utilizing on-chip vacuum packaging [24] or by employing nanomechanical resonators [25] . The use of nanomechanical resonators would also result in higher operation frequencies and integration densities, for example, a 1 GHz mechanical beam oscillator could be realized with a length and width of 1 μm and 100 nm, respectively, leading to integration densities as high as 10 8 oscillators per cm 2 (ref. 7 ). The outstanding obstacle in the realization of the above mechanical computer is a 1 GHz piezoelectric nanomechanical resonator with Q sufficiently high to yield good signal-to-noise ratios and the ability to host the parametric amplification functionality. A potential path to these requirements might be found via piezoelectric bulk acoustic wave resonators [26] . Whereas the performance of the current device is typically Δ ∼ 1 Hz per logic operation, it is instructive to estimate the prospects of this technology, for example, with a 1 GHz resonator with Q =100, yielding an operation bandwidth of 10 MHz (ref. 27 ). Using a state-of-the-art computer word size of 64 bits with 64 parallel processes would result in 5×10 6 64-bits logic operations per second with only a single nanomechanical device. If such nanomechanical processors were assembled on to a chip with the above described integration density, it could result in data-processing capacity of 10 14 Hz cm −2 . Even higher processing capacity would be available in graphene membrane resonators with dimensions of a few nanometers, in which resonance frequencies as high as 400 GHz could be achieved [28] . A nanomechanical computer realized in this mould would yield unprecedented data-processing power making it a highly tantalizing prospect, which merits further investigation. Experimental The electromechanical resonator was fabricated via conventional micromachining processes from a GaAs/AlGaAs modulation-doped heterostructure sustaining a 2DEG 90 nm below the surface. The sample was mounted in a high vacuum insert (8×10 −8 mbar), which was then placed in a 4 He cryostat at 3 K. The mechanical response was measured using standard low-frequency lock-in and amplification techniques. The signal, pump and reference (for the lock-in measurements) excitations were generated via six signal generators (NF Wavefactory 1974), which were coupled and synchronized via their internal 10 MHz reference clock. The electromechanical oscillator's response was amplified by an on-chip Si-nanofield-effect transistor with 30 dB gain, followed by a transimpedance amplifier (Femto DLPCA-200) with a gain of 10 7 VA −1 and measured in either a lock-in amplifier (Ametek 7265) or a spectrum analyser (Agilent 89410A). Multiple idler generation The mechanical oscillator response when injected with two detuned pumps with fixed frequency, f pA =2 f 0 +Δ and f pB =2 f 0 −Δ, while the system is also excited by f s = f 0 + δ is shown in Figure 2c . This measurement reveals a striking response from the mechanical oscillator with the observation of two first-order idlers two second-order idlers as well as two third-order idlers which arise because of the mixing of the pumps with first and second-order idlers ( Fig. 2d shows all the idlers marked). Moreover, by varying Δ, the idlers can be detuned around f 0 where larger values of Δ result in the higher order idlers becoming less visible as shown in Supplementary Figure S1c , that is, the idlers can only be observed within the bandwidth of the fundamental mode ( Supplementary Note 3 and Supplementary Figure S4 ). Numerical simulations The experimental measurements can be verified by simulating the response of the non-degenerate parametric oscillator with an equation of motion given by where x ( t ) is the resonator's position with damping γ =1/ Q and an effective spring constant containing a Duffing type nonlinearity parameterized by β and the parametric nonlinearity where Γ is the amplitude of the parametric modulation (pump) and Λ is the amplitude of the harmonic excitation (signal) where the signal and pump frequencies are given by Equation (4) is solved in the rotating frame at ω 0 by decomposing the resonator's position into in-phase and quadrature components where X ( t ) and Y ( t ) are slowly varying compared with ω 0 . Equation (4) can thus be expressed as Neglecting the off-resonance coefficients yields two first-order nonlinear differential equations Equation (9) can be readily modified to introduce n additional pumps as Additional signal excitations can also be introduced into equation (9) as where φ is the phase difference between the signal excitations s1 and s2. Equation (9) can be numerically solved using Euler's algorithm and the resulting amplitude at f 0 + δ is extracted by taking the Fourier transform F of X and Y as ( F ( X )− i F ( Y ))/2. Numerical simulations using this formulism can reproduce all the experimental results with β =0 and Γ=0.9γ, that is, just below the parametric resonance threshold where mixing between the signals and pumps is mediated by the parametric term (mixing mediated by the Duffing term, that is, β ≠0 is discussed in Supplementary Note 4 and is shown in Supplementary Figure S5 ). How to cite this article: Mahboob, I. et al . Interconnect-free parallel logic circuits in a single mechanical resonator. Nat. Commun. 2:198 doi: 10.1038/ncomms1201 (2011).